ELL facilitates RNA polymerase II pause site entry and release Transcription is a multi-stage process that coordinates several steps within the transcription cycle including chromatin reorganization, RNA polymerase II recruitment, initiation, promoter clearance and elongation. Recent advances have identified the super elongation complex, containing the eleven-nineteen lysine-rich leukaemia (ELL) protein, as a key regulator of transcriptional elongation. Here we show that ELL has a diverse and kinetically distinct role before its assembly into the super elongation complex by stabilizing Pol II recruitment/initiation and entry into the pause site. Loss of ELL destabilizes the pre-initiation complexes and results in disruption of early elongation and promoter proximal chromatin structure before recruitment of AFF4 and other super elongation complex components. These changes result in significantly reduced transcriptional activation of rapidly induced genes. Thus, ELL has an early and essential role during rapid high-amplitude gene expression that is required for both Pol II pause site entry and release. Transcription involves ordered assembly of transcriptional regulators and regulatory complexes that coordinate progressive changes in structure and activity of RNA polymerase II (Pol II), as it passes through the transcription cycle. These steps begin with the recruitment of Pol II to form the pre-initiation complex (PIC) through its assembly with general transcription factors and specific promoter proximal transcriptional co-regulators including the mediator complex [1] and the histone acetyl-transferase p300 (ref. 2 ), followed by transcription initiation, elongation, RNA processing, termination and export [3] . Although, for many years, the recruitment phase has been considered the major rate-determining step in transcription, recent studies show that Pol II is disproportionately accumulated in 'poised' or 'stalled states' at proximal promoters within 300 base pairs of the transcription start site of most mammalian and lower metazoan genes [4] , [5] , [6] , [7] . This widespread occurrence of proximally stalled Pol II has shifted the focus to understanding how transcriptional elongation is governed in complex organisms [8] . One component that has a central role in the release of Pol II from pausing is the positive transcriptional elongation factor b (P-TEFb), a heterodimeric kinase, composed of CDK9 and Cyclin T. P-TEFb, disables negative regulators of transcription and modifies Pol II at its Ser-2 carboxy-terminal domain (CTD) repeat by phosphorylation (pS2) to license assembly of multiple factors critical for mRNA biogenesis and chromatin modification during transcription [8] . A second well-known component is the ELL. ELL was first identified as a fusion partner of the MLL gene in chromosomal translocations associated with mixed lineage leukaemias in children [9] and shown later to increase elongation by reducing the rate of Pol II stalling during active transcription [10] . Recently, several groups have reported the in vitro identification of a higher order complexes containing ELL and P-TEFb in complex with multiple MLL translocation partners, including AFF1 (AF4), ENL , AF9 and AFF4 (AF5q31) [11] , [12] , [13] , [14] , [15] . The identification of this complex, referred to as the super elongation complexes (SECs), has highlighted the complexity of transcription and has led to several unifying concepts linking the control of transcriptional elongation to gene regulatory events central for cellular growth, development and leukaemogenesis [11] , [13] , [15] , [16] . More recently, several reports have characterized the formation and differential activity of ELL-containing subassemblies of the SEC complex, indicating that SEC assembly and function may be much more dynamic than previously believed [17] , [18] , [19] . In this study, by kinetically profiling the in vivo recruitment of ELL, RNA polymerase II, members of the PIC, and SEC components AFF4 and P-TEFb, we reveal a much earlier role for ELL in the transcription cycle before Pol II pause site entry. Reduction of endogenous ELL by gene depletion not only leads to reduced SEC assembly and P-TEFb recruitment, but results in destabilization and loss of Pol II and mediator components from the proximal promoter of rapidly induced genes during activated transcription. As a result, Pol II fails to enter the pause site, and there is attenuated accumulation of paused Pol II-associated short nascent RNA, and an accompanying redistribution of nucleosome density at the proximal promoter. Gene expression analysis demonstrates that ELL is broadly required for inducible transcriptional activation of many genes involved in stress and signal-regulated responses, including most immediate early genes. In contrast, depletion of the AFF4 SEC component produces much smaller influences on transcription than loss of ELL and does not significantly impair ELL recruitment, PIC assembly, or Pol II pause site entry. Finally, live cell imaging analysis of ELL and AFF4 loading at an endogenous gene array reveals that ELL and AFF4 load and reside at actively induced genes with different kinetics; therefore, they are likely to exist in multiple subassemblies distinct from a single large static complex. Together, these findings demonstrate that ELL has an essential and versatile role across many steps throughout the transcription cycle that are required to coordinate and synchronize the multiple rounds of PIC initiation/re-initiation with subsequent productive elongation, thus enabling rapid and high amplitude gene expression. ELL is required for rapidly induced transcription Several studies in different model systems have shown that ELL is required for Pol II Ser-2 CTD phosphorylation through its association with P-TEFb, and recent in vitro studies have revealed that this activity is linked to formation of the SEC through its co-assembly with AFF4 and AF9 family members [13] , [14] , [15] . However, the mechanism and dynamics of how ELL is recruited and functions to target these complexes to actively transcribing endogenous genes in mammalian cells is not clear. To begin to address these questions, we used a combination of gene expression, chromatin immunoprecipitation, and gene depletion strategies to profile ELL function at endogenous genes. By chromatin immunoprecipitation, the kinetic distribution of ELL within the promoter and transcribed regions of FOS and LDLR parallels the transcription of their respective mRNAs in mitogen (EGF)-induced HEK293 cells ( Fig. 1a,b ). ELL RNAi depletion results in global loss of both Pol II pS2 and elongation-associated histone H3K36Me3 tri-methylation ( Fig. 1c ). Notably, by microarray analysis, ELL gene depletion results in genome-wide loss of inducible expression of multiple genes involved in rapid stress and stimulus evoked gene expression in HEK293 cells ( Fig. 1c–e; Supplementary Table S1 ), including the immediate early genes FOS , LDLR , EGR2 and EGR3 ( Fig. 1f ). 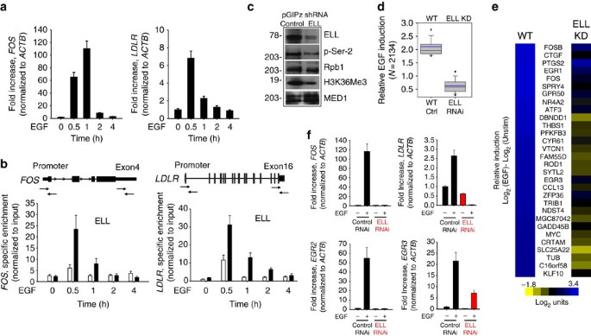Figure 1: ELL recruitment is required for rapidly induced gene expression. (a) Time course of EGF (50 ng ml−1)-induced expression ofFOSandLDLRby qRT–PCR in HEK293 cells. Error bars reflect the range of data formn=2 biological replicates. (b) SchematicFOSandLDLRloci with positions of ChIP primers and ELL ChIP profile of promoter and 3′ enrichment atFOSandLDLR.Error bars show the range of the data forn=2 biological replicates. (c) Immunoblot of ELL, Pol II pS2, total Pol II (Rpb1), histone H3K36Me3 tri-methylation and Med1 protein levels in control and cells depleted of ELL by RNAi. (d) Relative global EGF gene induction of control (WT) and HEK293 cells depleted of ELL by RNAi (ELL KD). Shown are comparison of topN=2134 genes that were induced >1.75-fold by EGF in control cells. Blue bar indicates mean, data points indicate 95th and 5th percentile. (e) Heat map of microarray analysis in (d) showing top 30 EGF-induced genes before and after ELL depletion. (f) qRT–PCR profiles ofFOS,LDLR,EGR2andEGR3transcription following EGF induction in control (black bars) and ELL-depleted HEK293 cells (red bars). Error bars show the range of data forn=2 biological replicates. Figure 1: ELL recruitment is required for rapidly induced gene expression. ( a ) Time course of EGF (50 ng ml −1 )-induced expression of FOS and LDLR by qRT–PCR in HEK293 cells. Error bars reflect the range of data form n =2 biological replicates. ( b ) Schematic FOS and LDLR loci with positions of ChIP primers and ELL ChIP profile of promoter and 3′ enrichment at FOS and LDLR. Error bars show the range of the data for n =2 biological replicates. ( c ) Immunoblot of ELL, Pol II pS2, total Pol II (Rpb1), histone H3K36Me3 tri-methylation and Med1 protein levels in control and cells depleted of ELL by RNAi. ( d ) Relative global EGF gene induction of control (WT) and HEK293 cells depleted of ELL by RNAi (ELL KD). Shown are comparison of top N =2134 genes that were induced >1.75-fold by EGF in control cells. Blue bar indicates mean, data points indicate 95th and 5th percentile. ( e ) Heat map of microarray analysis in ( d ) showing top 30 EGF-induced genes before and after ELL depletion. ( f ) qRT–PCR profiles of FOS , LDLR , EGR2 and EGR3 transcription following EGF induction in control (black bars) and ELL-depleted HEK293 cells (red bars). Error bars show the range of data for n =2 biological replicates. Full size image ELL recruits AFF4/P-TEFb complexes to rapidly induced genes A central observation that links MLL translocation partners to the regulation of transcriptional elongation during leukaemogenesis is their recursive interactions with each other and P-TEFb. This is supported by recent in vitro findings that complexes containing ELL, P-TEFb and the MLL translocation partner, AFF4, are stabilized by both Tat and CDK9 and can form a variety of stable intermediates with differential transcriptional activity [13] , [14] , [15] , [17] , [18] . The consensus from these biochemical studies is that AFF4 functions to 'scaffold' these interactions through contiguous amino-terminal domains that bind CDK9 (refs 11 , 12 , 14 , 16 , 20 ), CTDs that bind ELL [14] and recently recognized interactions between Cyclin T and ELL [17] . However, despite the observation that ELL, P-TEFb and AFF4 are capable of forming a holocomplex, the patterns of the assembly of these factors are not identical ( Fig. 2; Supplementary Fig. S1 ). Notably, the EGF-induced loading and distribution of ELL at the promoter and into the transcribed regions of immediate early genes shows relative enrichment in both regions ( Fig. 2 ). This pattern is significantly less prominent for P-TEFb ( Fig. 2 ) but consistent with its recruitment to the promoter by other transcription factors (for example, Myc, NF-kappa B, and Brd4 (refs 21 , 22 , 23 )). In contrast, mitogen-induced recruitment of AFF4 shows primarily progressive 3′ enrichment for AFF4 ( Fig. 2 ). The differences in these patterns suggest that ELL, P-TEFb and AFF4 may participate in separate assemblies before SEC formation. Nonetheless, in all cases, ELL depletion leads to significant loss of both P-TEFb and AFF4 recruitment following EGF induction ( Fig. 2 , black and white columns). 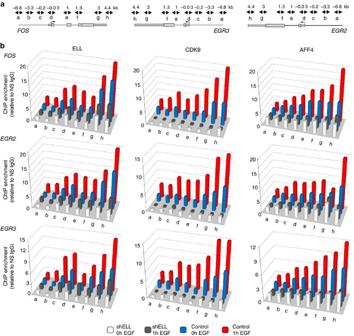Figure 2: ELL is required for recruitment of P-TEFb and AFF4. (a) Diagram of primer locations used for ChIP. (b) ChIP experiments showing ELL recruitment, P-TEFb (CDK9) recruitment, and AFF4 recruitment at theFOS,EGR2andEGR3genes following EGF induction (black and red bars) in wild-type HEK293 cells (red and blue bars) or cells depleted of ELL by RNAi (white and black bars). Average range of the error for each measurement is 15.3% of the mean forn=2 biological replicates. Figure 2: ELL is required for recruitment of P-TEFb and AFF4. ( a ) Diagram of primer locations used for ChIP. ( b ) ChIP experiments showing ELL recruitment, P-TEFb (CDK9) recruitment, and AFF4 recruitment at the FOS , EGR2 and EGR3 genes following EGF induction (black and red bars) in wild-type HEK293 cells (red and blue bars) or cells depleted of ELL by RNAi (white and black bars). Average range of the error for each measurement is 15.3% of the mean for n =2 biological replicates. Full size image ELL is required for PIC assembly and function Abrogated recruitment of SEC components P-TEFb and AFF4 after ELL depletion was expected. Surprisingly, however, ChIP studies of Pol II assembly, at immediate early genes, also reveal that PIC formation and subsequent CTD phosphorylation are also severely impaired by ELL depletion in EGF-stimulated cells ( Fig. 3 ; Supplementary Fig. S2 ). This significant decrease in the promoter proximal Pol II is readily evident by the paradoxical change in the pausing index [24] ( Fig. 3b , inset) in EGF-stimulated cells following ELL depletion. The absence of Pol II progression into the transcribed regions, accompanying Pol II (pS2) phosphorylation, and loading of the Cdk7 subunit of TFIIH ( Fig. 3 ) and Pol II serine 5 phosphorylation (pS5) ( Supplementary Fig. S3 ), indicate that ELL depletion produces a sweeping abrogation of Pol II recruitment and function, spanning multiple phases of PIC formation and early initiation during EGF induction of FOS , EGR2 and EGR3. 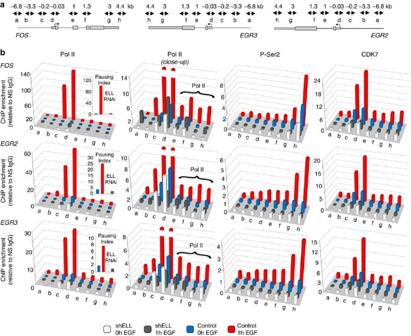Figure 3: ELL depletion results in destabilization and loss of Pol II from the proximal promoter of mitogen-induced genes. (a) Diagram of primer locations used for ChIP. (b) ChIP enrichment of Pol II, Pol II with close-up of transcribed region, Pol II CTD pS2 and CDK7 at the promoter and transcribed regions ofFOS,EGR2andEGR3, in resting (white and blue bars) or EGF-stimulated HEK293 cells (black and red bars) without (blue and red bars) and with ELL depletion by RNAi (white and black bars). Inset shows the Pol II pausing index in resting and EGF-stimulated cells before and after ELL depletion. Average range of the error for each measurement is 15.2% of the mean forn=2 biological replicates. Figure 3: ELL depletion results in destabilization and loss of Pol II from the proximal promoter of mitogen-induced genes. ( a ) Diagram of primer locations used for ChIP. ( b ) ChIP enrichment of Pol II, Pol II with close-up of transcribed region, Pol II CTD pS2 and CDK7 at the promoter and transcribed regions of FOS , EGR2 and EGR3 , in resting (white and blue bars) or EGF-stimulated HEK293 cells (black and red bars) without (blue and red bars) and with ELL depletion by RNAi (white and black bars). Inset shows the Pol II pausing index in resting and EGF-stimulated cells before and after ELL depletion. Average range of the error for each measurement is 15.2% of the mean for n =2 biological replicates. Full size image ELL forms distinct complexes with AFF4 and p300 The finding that ELL is required for both elongation factor recruitment and PIC formation suggests that ELL may interact with components of the PIC. In addition to ELL, prior studies have shown that p300 is also required for the activation of rapidly induced genes and both are rapidly recruited to gene promoter regions with similar kinetics [7] . Co-immunoprecipitation studies show that, in addition to Cdk9, ELL forms a direct complex with p300 in nuclear extracts from both resting and mitogen-induced cells ( Fig. 4a ). Moreover, cells depleted of p300 by RNAi ( Fig. 4b,c ) or by gene knockout ( Supplementary Fig. S4 ) show a major deficit in ELL recruitment following EGF stimulation, indicating a significant role for ELL/p300 interactions in ELL recruitment and stabilization of PIC assembly. In contrast, loss of ELL impairs neither p300 nor TBP recruitment ( Fig. 4c ), suggesting that ELL may assemble at later stages of PIC formation to stabilize the transition from initiation to early elongation during activated transcription. Consistent with this, glycerol gradient sedimentation analysis of nuclear extracts identifies separate populations of ELL co-migrating both with p300 as a smaller complex, and with AFF4 and other P-TEFb components as the larger SEC complex ( Fig. 4d; Supplementary Fig. S5 ). This interaction is demonstrated functionally by reporter assays, using a tethered Gal4–p300 fusion, to reveal that p300-driven transcriptional activation in the presence of CDK9 is highly synergistic with ELL ( Fig. 4e ). 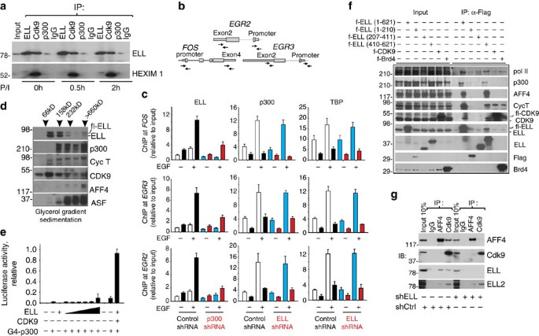Figure 4: ELL forms distinct complexes with p300 and AFF4. (a) Anti-ELL, anti-CDK9 and anti-p300 co-immunoprecipitation of ELL and HEXIM1 in Jurkat nuclear lysates at indicated time points following mitogen stimulation with phorbol ester and ionomycin (P/I). (b) Diagram of primer locations used for ChIP. (c) ChIP profile of ELL, p300 and TBP association with promoter (white and blue bars) and transcribed regions (black and red bars) of theFOS,EGR3andEGR2genes in resting or EGF-stimulated control (white and black bars) and p300-depleted HEK293 cells or ELL-depleted HEK293 cells (blue and red bars), as indicated. Error bars show the range of error forn=2 biological replicates. (d) ELL, p300, CycT1, CDK9, AFF4, and ASF/SF2 immunoblot profiles of 10–40% glycerol density gradient sedimentation of nuclear lysates of HEK293 cells stably expressing Flag-ELL. Every third fraction was analysed. Approximate positions from top (left) to bottom (right) of molecular weight markers are shown. (e) Gal4–p300 reporter assay in HEK293 cells co-transfected with combinations of ELL (50–1,000 ng), Gal4–p300 fusion protein (500 ng), and CDK9 (1 μg) expression vectors normalized to percent of maximum signal. Error bars represent the range of the data forn=2 independent biological replicates. (f) Anti-Flag co-immunoprecipitation experiments of endogenous RNAPII (Pol II), p300, AFF4, CycT, CDK9, and BRD4 in HEK293 cells expressing Flag epitope tagged ELL and ELL truncation mutant. (g) Reciprocal immunoprecipitation of AFF4, CDK9, ELL and ELL2 by AFF4 and CDK9 antibodies before and after ELL depletion by RNAi. Figure 4: ELL forms distinct complexes with p300 and AFF4. ( a ) Anti-ELL, anti-CDK9 and anti-p300 co-immunoprecipitation of ELL and HEXIM1 in Jurkat nuclear lysates at indicated time points following mitogen stimulation with phorbol ester and ionomycin (P/I). ( b ) Diagram of primer locations used for ChIP. ( c ) ChIP profile of ELL, p300 and TBP association with promoter (white and blue bars) and transcribed regions (black and red bars) of the FOS , EGR3 and EGR2 genes in resting or EGF-stimulated control (white and black bars) and p300-depleted HEK293 cells or ELL-depleted HEK293 cells (blue and red bars), as indicated. Error bars show the range of error for n =2 biological replicates. ( d ) ELL, p300, CycT1, CDK9, AFF4, and ASF/SF2 immunoblot profiles of 10–40% glycerol density gradient sedimentation of nuclear lysates of HEK293 cells stably expressing Flag-ELL. Every third fraction was analysed. Approximate positions from top (left) to bottom (right) of molecular weight markers are shown. ( e ) Gal4–p300 reporter assay in HEK293 cells co-transfected with combinations of ELL (50–1,000 ng), Gal4–p300 fusion protein (500 ng), and CDK9 (1 μg) expression vectors normalized to percent of maximum signal. Error bars represent the range of the data for n =2 independent biological replicates. ( f ) Anti-Flag co-immunoprecipitation experiments of endogenous RNAPII (Pol II), p300, AFF4, CycT, CDK9, and BRD4 in HEK293 cells expressing Flag epitope tagged ELL and ELL truncation mutant. ( g ) Reciprocal immunoprecipitation of AFF4, CDK9, ELL and ELL2 by AFF4 and CDK9 antibodies before and after ELL depletion by RNAi. Full size image We used domain-dependent profiling to gain further insight into the multiple interactions coordinated between ELL and components of the PIC and SEC ( Fig. 4f; Supplementary Fig. S6 ). Epitope-tagged truncation mutants of ELL reveal that, although multiple domains of ELL, including the N-terminal (1–210 aa), mid-portion (207–411aa) and C-terminal (410–621) domains, are capable of interacting with Pol II, only the C-terminal ELL domain, or full length ELL form complexes with p300, P-TEFb and AFF4 ( Fig. 4f ). Prior studies have shown that the bromodomain protein Brd4 also interacts with P-TEFb to target it to active genes [7] , [25] . However, although both ELL and Brd4 are avidly co-recruited to active promoters [7] , they appear to form independent complexes in cellular extracts ( Fig. 4f; Supplementary Fig. S5 ), as has been suggested by prior studies [14] , [15] . Finally, although recent studies have regarded ELL and its ELL2 paralogue as interchangeable, the nature of their interaction or whether they assemble in the same complex remains unclear [13] , [14] , [19] , [26] . Immunoprecipitation of endogenous complexes in cells depleted of ELL reveals a significant role for ELL in maintaining the integrity of the SEC complex bacause its depletion reduces the levels of AFF4 associated with immunoprecipitated CDK9 ( Fig. 4g ). Even though the ELL2 paralogue readily forms complexes with AFF4, its levels do not compensate for ELL depletion; thus, ELL2-containing complexes seem to assemble independent of ELL ( Fig. 4g ). ELL facilitates recruitment of PIC mediator components Rapid high-amplitude transcription requires that the re-initiation complex assembles quickly and efficiently. The residual PIC components that remain following Pol II promoter escape is referred to as the scaffold PIC, and the mediator complex has a central role in its stability and function [1] , [27] . Consistent with its requirement for PIC stability, cells depleted of ELL show a marked decrease in both Med 1 and CDK8 mediator components following EGF stimulation ( Fig. 5a,b; Supplementary Fig. S7 ). Thus, multiple dynamic members of the PIC assembly, including components of mediator thought to facilitate rapid transition to elongation (CDK8) [28] , show impaired recruitment to actively induced genes in the absence of ELL. 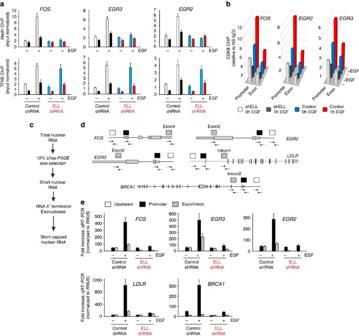Figure 5: ELL is required in post-recruitment steps before commitment to productive elongation. (a) ChIP enrichment of Med1 and TFIIB at the promoter (white and blue bars) and transcribed regions (black and red bars) of theFOS,EGR3, andEGR2genes in resting or EGF-stimulated HEK293 cells before (white and black bars) and after ELL depletion by RNAi (blue and red bars). Error bars show the range of error forn=2 biological replicates. (b) ChIP enrichment of CDK8 at the promoter and transcribed regions of theFOS,EGR3andEGR2genes in resting (grey and blue bars) or EGF-stimulated (black and red bars) HEK293 cells before (blue and red bars) and after ELL depletion by RNAi (white and black bars). Average range of error is 14.7 % of the mean fromn=2 biological replicates. (c) Experimental scheme for short nascent RNA detection. (d) Schematic of primer location for detection of profiles of short nascent RNA from theFOS,EGR3,EGR2,LDLRandBRCA1genes. White bar indicates regions upstream of the promoter. Black bars indicate promoter regions. Grey bars indicated downstream intron/exon regions. (e) Profile of short nascent RNA fromFOS,EGR3,EGR2,LDLRandBRCA1genes in resting and EGF-stimulated HEK293 cells before and after ELL depletion by RNAi. Levels were normalized toRNU5RNA. Error bars show the range of error forn=2 biological replicates. Figure 5: ELL is required in post-recruitment steps before commitment to productive elongation. ( a ) ChIP enrichment of Med1 and TFIIB at the promoter (white and blue bars) and transcribed regions (black and red bars) of the FOS , EGR3 , and EGR2 genes in resting or EGF-stimulated HEK293 cells before (white and black bars) and after ELL depletion by RNAi (blue and red bars). Error bars show the range of error for n =2 biological replicates. ( b ) ChIP enrichment of CDK8 at the promoter and transcribed regions of the FOS , EGR3 and EGR2 genes in resting (grey and blue bars) or EGF-stimulated (black and red bars) HEK293 cells before (blue and red bars) and after ELL depletion by RNAi (white and black bars). Average range of error is 14.7 % of the mean from n =2 biological replicates. ( c ) Experimental scheme for short nascent RNA detection. ( d ) Schematic of primer location for detection of profiles of short nascent RNA from the FOS , EGR3 , EGR2 , LDLR and BRCA1 genes. White bar indicates regions upstream of the promoter. Black bars indicate promoter regions. Grey bars indicated downstream intron/exon regions. ( e ) Profile of short nascent RNA from FOS , EGR3 , EGR2 , LDLR and BRCA1 genes in resting and EGF-stimulated HEK293 cells before and after ELL depletion by RNAi. Levels were normalized to RNU5 RNA. Error bars show the range of error for n =2 biological replicates. Full size image ELL is required for promoter clearance and pause site entry Recent genome-wide studies have shown that Pol II pausing and abortive elongation are often associated with accumulation of short-capped nascent RNA transcripts generated by stalled polymerases [5] . To test whether ELL is required for events during early elongation, the levels of short-capped nascent RNAs were detected using the method described by Nechaev et al . [5] ( Fig. 5c ). Strikingly, loss of ELL results in a significant decrease in the formation of short-capped RNAs during mitogen induction of FOS , EGR3 , EGR2 , LDLR and BRCA1 ( Fig. 5d-e ). These observations support the finding that ELL is required during early elongation in a manner that is distinct from its role in releasing Pol II from stalling by recruitment of P-TEFb and AFF4 ( Fig. 2 ) [13] , [14] , [15] . ELL exists in functional complexes independent of AFF4 The early function for ELL in promoter clearance and pause site entry is in distinct contrast to the much later sequential role AFF4 had. AFF4 depletion shows little influence on the accumulation of nascent-capped short RNA transcripts following mitogen induction ( Fig. 6a,b ). Consistent with this observation, AFF4 depletion shows modest effects on P-TEFb recruitment and insignificant influence on ELL recruitment at FOS , EGR3 and EGR2 ( Fig. 6c ). Accordingly, AFF4 depletion is much less effective in decreasing transcription of FOS , EGR3 , EGR2 , LDLR, JUN and BRCA1 ( Fig. 6d ) in comparison to depletion of ELL ( Fig. 1f ). Finally, live cell imaging of GFP-tagged AFF4 and ELL loading at the MMTV array [29] in glucocorticoid-stimulated cells reveal different fluorescent recovery after photobleaching (FRAP) profiles demonstrating that ELL and AFF4 do not exist exclusively in a single static complex and are, therefore, likely to have both overlapping and distinct roles throughout the transcription cycle ( Fig. 6e ). 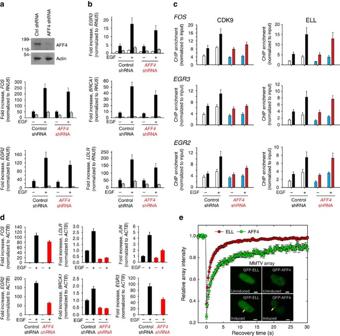Figure 6: AFF4 is not required at early steps in the transcription cycle. (a) Immunoblot of AFF4 expression in control and AFF4 shRNA expressing cells. (b) Short nascent RNA profile ofFOS, EGR2, EGR3, LDLRandBRCA1genes in resting and EGF-stimulated cells before and after AFF4 depletion by RNAi. White bars indicate regions upstream of the promoter. Black bars indicate promote regions. Grey bars indicated downstream intron/exon regions. (c) ChIP profile of ELL recruitment and CDK9 recruitment to the promoter (white and blue bars) and transcribed regions (black and red bars) ofFOS,EGR3, andEGR2in resting and EGF-stimulated HEK293 cells before (white and black bars) and after AFF4 depletion by RNAi (blue and red bars). Error bars show the range of error forn=2 biological replicates. (d)FOS,EGR2,LDLR,BRCA1,JUNandEGR3expression in resting and EGF-stimulated cells before (black bars) and after AFF4 depletion by RNAi (red bars). Error bars show the range of error forn=2 biological replicates. (e) GFP-tagged AFF4 and ELL FRAP recovery at MMTV array in glucocorticoid stimulated 3134 cells. Error bars, s.d. ofn=17 (AFF4-GFP) andn=11 (ELL-GFP) biological replicates. Scale bar, 5 μν Figure 6: AFF4 is not required at early steps in the transcription cycle. ( a ) Immunoblot of AFF4 expression in control and AFF4 shRNA expressing cells. ( b ) Short nascent RNA profile of FOS, EGR2, EGR3, LDLR and BRCA1 genes in resting and EGF-stimulated cells before and after AFF4 depletion by RNAi. White bars indicate regions upstream of the promoter. Black bars indicate promote regions. Grey bars indicated downstream intron/exon regions. ( c ) ChIP profile of ELL recruitment and CDK9 recruitment to the promoter (white and blue bars) and transcribed regions (black and red bars) of FOS , EGR3 , and EGR2 in resting and EGF-stimulated HEK293 cells before (white and black bars) and after AFF4 depletion by RNAi (blue and red bars). Error bars show the range of error for n =2 biological replicates. ( d ) FOS , EGR2 , LDLR , BRCA1 , JUN and EGR3 expression in resting and EGF-stimulated cells before (black bars) and after AFF4 depletion by RNAi (red bars). Error bars show the range of error for n =2 biological replicates. ( e ) GFP-tagged AFF4 and ELL FRAP recovery at MMTV array in glucocorticoid stimulated 3134 cells. Error bars, s.d. of n =17 (AFF4-GFP) and n =11 (ELL-GFP) biological replicates. Scale bar, 5 μν Full size image ELL loss disrupts local histone density and modifications To assess whether or not depletion of ELL can influence histone marks and nucleosomal structure at mitogen-inducible genes, the distribution of total histone, the activation-associated histone H3K4Me3 tri-methylation mark and the elongation-associated histone H3K36Me3 tri-methylation mark were profiled across the promoter and transcribed regions of FOS , EGR3 and EGR2 in cells depleted of ELL before mitogen stimulation ( Fig. 7 ; Supplementary Fig. S8 ). As demonstrated in Fig. 7 , loss of ELL results in depletion of histone H3K4Me3 activation marks at the proximal promoter of mitogen-induced genes, and this reduction is associated with an increase in total histone 4 densities within the proximal promoter, suggesting the licensing of a more repressive chromatin state in the absence of ELL. In addition, and consistent with the role of ELL as an elongation factor, the elongation-associated histone H3K36Me3 tri-methylation marks are significantly repressed in the absence of ELL ( Fig. 7 ). Notably, this redistribution resembles other cellular systems in which the paused or promoter proximal RNA polymerase II is destabilized [30] , [31] , [32] . 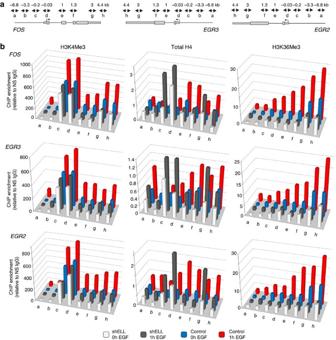Figure 7: Loss of ELL leads to disruption of chromatin marks and histone distribution at mitogen-induced genes. (a) Schematic of gene loci showing positions of ChIP primers used in the study. (b) ChIP profile of histone H3K4Me3 tri-methylation, total histone 4 distribution, and histone H3K36Me3 tri-methylation atFOS,EGR3andEGR2in resting (white and blue) and EGF-stimulated (black and red) HEK293 cells before (blue and red) and after (white and black) ELL depletion by RNAi. Average range of the error for each measurement is 16.8 % of the mean forn=2 biological replicates. Figure 7: Loss of ELL leads to disruption of chromatin marks and histone distribution at mitogen-induced genes. ( a ) Schematic of gene loci showing positions of ChIP primers used in the study. ( b ) ChIP profile of histone H3K4Me3 tri-methylation, total histone 4 distribution, and histone H3K36Me3 tri-methylation at FOS , EGR3 and EGR2 in resting (white and blue) and EGF-stimulated (black and red) HEK293 cells before (blue and red) and after (white and black) ELL depletion by RNAi. Average range of the error for each measurement is 16.8 % of the mean for n =2 biological replicates. Full size image In this study, we show that ELL has multiple distinct roles in the hierarchy of transcriptional events leading to production of mature RNA transcripts. These functional roles, in processes that span both early and late transcriptional events, are reminiscent of the ability of TFIIF and TFIIS to control steps in both transcriptional initiation and elongation [3] , [33] . One of the most interesting findings in this study is the early role of ELL in stabilizing the re-initiation complex and early elongation. This step is very distinct from its later role in recruiting P-TEFb and other SEC-associated complexes to the elongating polymerase and suggests that ELL, like TFIIF and TFIIS, may actively shuttle between different transcriptional states of Pol II (refs 3 , 34 ). It is noteworthy that these findings are not incompatible with the in vitro detection of ELL in large molecular weight complexes [13] , [15] , but rather serve to illustrate that the assembly of these transcriptional complexes is likely to be a highly dynamic, rather than static, process. Thus, it is more feasible that in vivo higher order complexes containing ELL assemble sequentially and dynamically at endogenous genes rather than engaging promoters as pre-assembled 'supercomplexes'. Therefore, our findings are consistent with a molecular scenario in which ELL assembles first with the initiating polymerase at the proximal promoter, where it helps to establish interactions between Pol II, mediator and p300 during early elongation. This step serves both to stabilize the re-initiation complex for subsequent rounds of transcription, and to later position ELL so that it can act as a platform to enable the subsequent recruitment of P-TEFb and AFF4 to the pre-elongation complex ( Fig. 8 ). This sequential model is consistent with the finding that early elongation is impaired by loss of ELL but not AFF4. 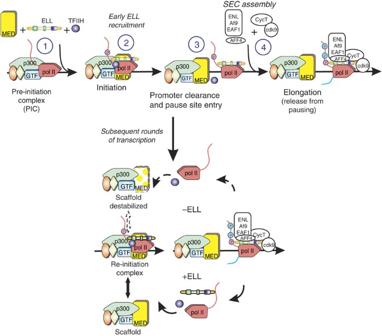Figure 8: Model for sequential loading of ELL. Schematic diagram of ELL recruitment to the PIC before loading of other components containing AFF4, P-TEFb, ENL, Af9 and EAF1 to assemble the SEC; and its subsequent recycling to support multiple rounds of transcription re-initiation (figure is adapted from Fudaet al.42). Figure 8: Model for sequential loading of ELL. Schematic diagram of ELL recruitment to the PIC before loading of other components containing AFF4, P-TEFb, ENL, Af9 and EAF1 to assemble the SEC; and its subsequent recycling to support multiple rounds of transcription re-initiation (figure is adapted from Fuda et al . [42] ). Full size image An extra novel finding in this study is a possible role for ELL in stabilizing recruitment and assembly of the Med1 component of mediator. These findings are highly consistent with recent observation that the Med26 component of the mediator complex can function to recruit ELL/EAF containing complexes to the PIC complex [18] . Similar to the study by Biswas et al ., [17] this study also suggested that there may be multiple ELL containing complexes that have differential functional activity [18] . Notably, the differential function of ELL-containing complexes separate from AFF4 is suggested in recent genome-wide profiling in mouse embryonic stem cells that show a distinct and separate peak for AFF4 downstream of ELL2 (ref. 19 ). Which mechanisms and kinetics underlie this activity at both the PIC and re-initiation complex of rapidly induced endogenous genes will require extensive future investigation. It is important to note that Med1 is a very dynamic component of the mediator complex that interacts with a variety of transcription factors and nuclear hormone receptors and is a target for mitogen-induced post-translational modification [35] . Thus, the potential for the regulation of ELL interaction with the PIC complex by a variety of signalling pathways is enormous. Finally, recent studies by Biswas et al . also suggest that other components of SEC like AF9 may also have roles at earlier stages of transcription [17] . Therefore, ELL is not likely to be the only member of the SEC complex with multiple distinct roles across the transcription cycle. Clearly, a lot remains to be understood about this new function for ELL in the transcription cycle and, by association, the differential role of mediator and SEC components during early elongation. The finding that loss of ELL, like loss of NELF, results in destabilization of promoter proximal Pol II, and a shift of histone density into the proximal promoter is very provocative, and suggest that, depending on promoter context, NELF may have a more positive role in enhancing transcription by stabilizing the PIC at points of transition to early elongation. It should be noted that loss of ELL also reduces recruitment of NELF to the proximal promoter of mitogen-induced genes (J.S.B., unpublished observation). Nonetheless, further kinetic studies will be needed to dissect the precise dynamics of this interaction. The discovery and identification of the web of interactions demonstrated by MLL fusion partners has generated new insights into understanding the regulation of transcriptional elongation; however, more needs to be learned about the mechanisms governing how different MLL translocation partners are assembled at genes in physiological and leukaemic backgrounds and what their true molecular functions are at endogenous genes. The finding that ELL has roles much earlier in the transcription cycle suggests that the mechanism of action of MLL translocation partners may be more divergent and stratified than previously perceived. Each leukaemogenic MLL fusion may have particular molecular features and factor dependencies that will prove highly relevant for future exploitation in molecular treatment strategies tailored to individual MLL translocation partners. Notably, the finding that ELL also interacts with p300, another well-known translocation partner of MLL in MLL leukaemias [36] confirms the existence of yet another node in the 'MLL web' [37] of interactions. Finally, the global gene expression profiling suggests an essential role for ELL in the expression of rapidly induced genes to facilitate quick responses to environmental cues. Interestingly, this parallels the recently uncovered positive role for CKD8 at immediately early genes [28] , thus suggesting a selective interaction between ELL and CDK8-containing mediator complexes during such events. In any regard, these are precisely the type of cellular programmes that were predicted to require or utilize paused polymerases to enable rapid response from 'poised' states. Although this trend was first uncovered in earlier genome-wide studies of paused polymerases [38] , [39] , it highlights the potential role for ELL in developmentally regulated gene expression programs at multiple steps throughout the loading and release of productively elongating Pol II at targeted genes. Cell lines and transfection Jurkat T and HEK293 cells were grown in RPMI medium supplemented with 10% FCS and 100 U ml −1 penicillin and streptomycin (Invitrogen) in a humidified atmosphere at 37 °C with 5% CO 2 (ref. 7 ). Plasmids expressing each Flag epitope-tagged ELL (f-ELL1-621), ELL truncation mutants (ELL1-210; ELL207-411; ELL410-621), and Brd4 (f-Brd4) were used [23] , [40] . Vectors expressing Flag-tagged CDK9 were generously provided by Dr Sergei Nekhai (Howard University). Transfections were performed using Lipofectamine 2000 (Invitrogen) according to the manufacturer's instructions. The EGFP–ELL (GFP–ELL) and EGFP–AFF4 (GFP–AFF4) constructs were generated by ligating ELL and AFF4 cDNA (OriGene) into a pEGFP-C2 (Clontech) vector as EcoRI-KpnI and XhoI-BamHI fragments, respectively. The pE-Cherry-FP-C1-GR construct was generously provided by Gordon Hager, National Cancer Institute, Bethesda. The 3134 cell line is a subclone of 904.13 derived from a mouse mammary adenocarcinoma cell line, C127 and harbours a large tandem array of ∼ 200 copies of the mouse mammary tumour virus promoter driving Ha- v-ras expression in a head-to-tail orientation [29] provided by Gordon Hager, National Cancer Institute, Bethesda. Immunoprecipitation and glycerol gradient sedimentation Immunoprecipitation was carried out with 10 8 Jurkat cells for each condition (control and stimulated with 50 ng ml −1 PMA and 1 μM Ionomycin as indicated) or 2×10 6 HEK293 transfected with Flag-tagged expression vectors. Nuclear extracts and whole cell lysates were generated as described previously [41] . Glycerol ultracentrifugation (Beckmann SW 60Ti, 20 h at 272,400×g) was performed as previously described [23] . Nuclei (2×10 8 cells), isolated by the method of Dignam and Roeder, were sonicated at 4 °C (Diagenode Bioruptor, 6 cycles on 6 cycles off) in buffers containing 10 mM HEPES, pH 7.9, 200 mM KCl, 1.5 mM MgCl 2 , 0.2 mM EDTA and 4 mM beta-mercaptoethanol, and clarified by centrifugation at 100,000 g for 30 min at 4 °C, before loading onto 10–40% glycerol gradients. Antibody conditions used for immunoprecipitation and western blotting are provided in Supplementary Table S2 . Chromatin immunoprecipitation and RNAi HEK293 wild-type (WT) and ELL KD cells were stimulated with EGF (50 ng ml −1 ) (Peprotech) for 1 hr, fixed 5 min in 1% formaldehyde at 4 °C, quenched and collectted for chromatin immunoprecipitation. The cross-linked cell pellets (1×10 7 ) were thawed on ice, resuspended in 1 ml of low-salt IP buffer (150 mM NaCl, 50 mM Tris–HCl (pH 7.5), 5 mM EDTA, 0.5% Nonidet P-40, and 1% Triton X-100) with 1× protease inhibitor mixture (Sigma-Aldrich), and sonicated for 4 min (20 s 'on' and 30 s 'off') at 3.0 power output using a Misonix Sonicator 3000 (Misonix) [7] . Total RNA was prepared using the Qiagen RNAeasy Kit following the manufacturer's instructions. RT reactions were performed with Omniscript (Qiagen) following the standard protocol [7] . (Primers used are provided in the Supplementary Materials ). For RNAi studies, transfections were performed in 6 wells and 10-cm culture vessels using plasmids expressing ELL- and AFF4-specific shRNA (Open Biosystem). HEK293 cells (6.0×10 5 in 6 wells and 5×10 6 ) were transfected with ELL shRNA and Lipofectamine 2000 reagent with varying concentrations (4 and 8 μg) of plasmid DNA and the ratio of DNA and Lipofectamine 2000 (1:0.5 to 1:5). Non-targeting pGIPz shRNA was used as a control. Antibodies and primers used for the analysis are provided in Supplementary Tables S2–S4 . Gene expression microarray Total RNA from unstimulated WT and ELL KD HEK293 and stimulated (EGF, 50 ng ml −1 ) WT and ELL KD HEK293 cells were isolated and purified using the Qiagen RNAeasy Kit following the manufacturer's instructions 7 and submitted to LMT-Affymetrix microarray facility to obtain the raw data (NCI-Frederick). The microarray data has been deposited in the GEO database under the GSE34104. Expression profiling by Affymetrix exon microarray analysis Affymetrix Human Exon ST1.0 platform was used for the microarray analysis. Raw data in CEL files were preprocessed using Affymetrix Expression Console software with 'RMA polish/RMA' option and its median normalization method. 'Core' confidence was used for the exon annotation. We profiled expression of each sample in biological duplicates. The exon-level value was taken to be the average of the two biological replicates. The gene-level expression value was obtained by taking the mean of the two exons with the highest signal intensity for the transcript. Preparation and detection of short-capped RNA The total RNA from HEK293 WT and ELL KD cells after transfection were isolated with ZR RNA MiniPrep (ZYMO Research). Short RNAs (50–250bp) were purified on 15% TBE UREA gel (Invitrogen) and recovered with ZR small-RNA PAGE Recovery Kit (Invitrogen). Purified short RNA was treated with the Terminator 5′-Phosphate-Dependent Exonuclease to remove uncapped 5′ RNA and then reverse transcribed to produce the cDNA with Quantitect Reverse Transcription Kit (QIAGEN). RNU5 was used as a loading control for quantitative PCR. Primer used for the analysis are provided in Supplementary Table S5 . Live-cell imaging and FRAP Before live-cell imaging, 3134 cells were plated in coverglass bottom chambers (Lab-Tek) containing Phenol Red-free RPMI (Gibco BRL) supplemented with 10% charcoal-stripped fetal bovine serum (Atlanta Biologicals). The 3134 cells were transiently co-transfected using Lipofectamine 2000 according to the manufacturer's protocol (Invitrogen) to express mCherry-GR and either EGFP–ELL or EGFP–AFF4. The 3134 cells transiently expressing both mCherry-GR and either EGFP–ELL or EGFP–AFF4 were treated with 100 nM dexamethasone (Sigma) for 20 minutes. Imaging and FRAP experiments were performed using a Zeiss LSM 5 Live Confocal Duoscan microscope with a ×63/1.4 oil immersion objective enclosed in a 5% CO 2 and 37 °C humidified chamber. Identification of MMTV arrays marked by the localization of mCherry-GR was achieved by exciting Cherry in the cells with the 561-nm 40-mW diode-pumped solid-state laser at 3% power. The mCherry emission was monitored with a LP 580 filter. Localization of EGFP–ELL or EGFP–AFF4 to the MMTV array was identified by exciting EGFP in the cells with the 488-nm 100-mW diode laser at 6% power. EGFP emission was monitored with a BP 495–555 filter. A nuclear region of interest containing the array was bleached with the 488 nm laser at 100% power. A single iteration was used for the bleach pulse lasting ∼ 0.025 seconds. EGFP–ELL or EGFP–AFF4 was monitored every 0.250 s for 75 s with the 488 nm laser 6 % power to minimize photobleaching. Image series were included with 50 pre-bleach images for normalization of data. All FRAP curves were then normalized and averaged to generate an overall FRAP curve. Acccession codes: the microarray data has been deposited in the GEO database under the GSE34104 . How to cite this article: Byun, J.S. et al . ELL facilitates RNA polymerase II pause site entry and release. Nat. Commun. 3:633 doi: 10.1038/ncomms1652 (2012).